Dynamic haematopoietic cell contribution to the developing and adult epicardium The epicardium is a cellular source with the potential to reconstitute lost cardiovascular tissue following myocardial infarction. Here we show that the adult epicardium contains a population of CD45+ haematopoietic cells (HCs), which are located proximal to coronary vessels and encased by extracellular matrix (ECM). This complex tertiary structure is established during the regenerative window between post-natal days 1 and 7. We show that these HCs proliferate within the first 24 h and are released between days 2 and 7 after myocardial infarction. The ECM subsequently reforms to encapsulate HCs after 21 days. Vav1-tdTomato labelling reveals an integral contribution of CD45+ HCs to the developing epicardium, which is not derived from the proepicardial organ. Transplantation experiments with either whole bone marrow or a Vav1+ subpopulation of cells confirm a contribution of HCs to the intact adult epicardium, which is elevated during the first 24 weeks of adult life but depleted in aged mice. In the adult mammalian heart, the existence of resident stem cells, which can act to restore lost tissue after a heart attack (myocardial infarction (MI)) [1] , is the subject of ongoing investigation. The adult epicardium, classically described as a single cell layer epithelium (mesothelium) lining the chamber myocardium of the heart, has emerged in recent times as a putative resident source of cardiovascular progenitors, which when appropriately activated, for example, by pharmacological treatment with factors such as thymosin β4, can contribute to neovascularisation and myocardial regeneration of the injured adult mouse heart [2] , [3] . In addition, the adult epicardium also acts as an important source of trophic signals and has been shown to secrete a number of key angiogenic signals to instruct new coronary vessel growth following MI [4] . The application of epicardial cell biology to the treatment of cardiovascular injury originates from the epicardium’s developmental potential and from the ability to reactivate these properties in the adult heart. During heart development, the epicardium arises from a transient structure called the proepicardial organ (PEO), of mesoderm origin, located at the inflow region of the developing heart tube above the primordial liver (reviewed in ref. 5 ). As the heart begins to loop (E8.5–9.0 in mouse), PEO cells undergo epithelial–mesenchymal transition to migrate towards the developing myocardium and envelop it to form the epicardium proper. This is then followed by a successive round of epithelial–mesenchymal transition, whereby epicardium-derived cells (EPDCs) migrate into the sub-epicardial region and contribute interstitial fibroblasts, vascular smooth muscle cells and, to a lesser extent, coronary endothelial cells and cardiomyocytes to the embryonic heart. The retained fetal epicardial layer also provides growth factors and cytokines to nurture the growth of the underlying myocardium (reviewed in ref. 6 ). A re-expression of embryonic epicardial genes (characterized by the signature genes Wt1 , Tbx18 and Raldh2 ) initiates adult EPDC activation [3] , [4] and is a hallmark of the downstream contribution of EPDCs in response to MI. The plasticity of EPDCs in the injury setting [2] , [3] , [4] , [7] prompted us to investigate whether the adult epicardium might be a more complex structure than the previously described simple mesothelium, and whether it might house heterogeneous cell types to act as a regenerative reserve during cardiovascular homeostasis and in response to stress or pathology. Thus far, the potential of the adult epicardium to be reactivated and contribute to cardiac repair has been realized entirely in the context of reactivation of a dormant, homogeneous single epithelial cell layer. Our findings suggest the epicardium is not a simple mesothelium but is, in fact, made up of discrete clusters of heterogeneous cell types, which include a novel haematopoietic contribution of distinct origin, encased by extracellular matrix (ECM) that anatomically resembles a stem or progenitor cell ‘niche’. This establishes the basis for a re-evaluation of the reparative potential of the adult epicardial lineage. Moreover, a haematopoietic cell (HC) contribution to the epicardium during development and adult homeostasis contrasts with the canonical view of a single PEO source maintained in steady state throughout adulthood. Consequently, the complex architecture of the adult epicardium and turnover of diverse constituent cell types offers the possibility of pharmacological targeting in cardiovascular repair. Adult epicardial cell clusters encased by extracellular matrix We first analysed intact hearts and, contrary to the prevailing view of the epicardium as a single cell layer, observed small cells with large nuclei-cytoplasmic ratios in situ , at intervals throughout the ventricular chambers and contiguous with the epicardium, as defined by the surface glycoprotein podoplanin [3] ( Fig. 1a–c ). These cell clusters were held in suspension via basement membrane proteins and key components of the ECM such as fibronectin ( Fig. 1d,e ; Supplementary Fig. 1a–f ), β1-integrin (CD29; Fig. 1f ), collagen IV ( Supplementary Movie 1 of a confocal Z -stack projection) and hyaluronic acid ( Supplementary Fig. 1g–r ). The cells within these apparent ‘microenvironments’ contained a population defined by specific expression of the cell surface glycoprotein CD44 (ref. 8 ), previously shown to mark a population of PEO origin that was proposed to give rise to mesenchymal-like stem cells residing within the adult epicardium [9] ( Fig. 1g ). Further characterization revealed the presence of distinct CD45+ HCs ( Fig. 1h ), which represented the more predominant resident population. Epicardium cell clusters were localized in close proximity to superficial coronary vessels ( Fig. 1i,j ), including those that contained CD45+ HCs ( Fig. 1k ). Each cluster consisted of between 3 and 15 CD45+ cells; the mean number of cells per cluster was 6.6±1.8 s.e.m. ( n =25 sections across 5 hearts, at 8 weeks of age) and there were 2.12±0.26 clusters per mm of epicardium (mean circumference of epicardium/total number of cell clusters/section±s.e.m. ; n =25 sections analysed across 5 hearts, at 8 weeks of age; P <0.01; Student's t -test). These data suggest the epicardium is not a simple mesothelium [10] , but contains structures that represent a heterogeneous mix of cell populations, including HCs, with vascular support and a non-cellular contribution of ECM. 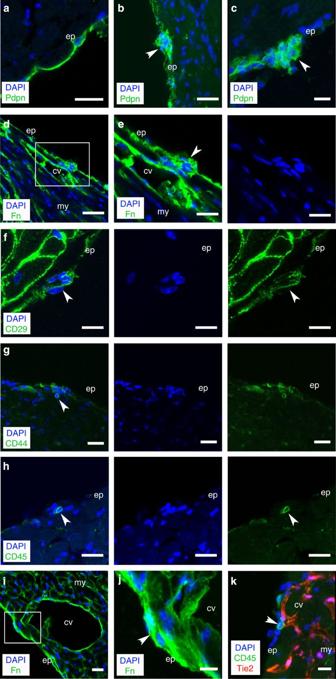Figure 1: Clusters of cells constrained by ECM exist in the intact adult epicardium. Immunofluorescent staining (IMF) for podoplanin (Pdpn; green) in the intact adult epicardium identifies clusters of cells within basement membrane (white arrowheads;a–c). Clusters in the epicardium (white arrowheads) are encapsulated by ECM as indicated by IMF for fibronectin (Fn; green;d). Inset box indis shown at higher magnification ine, and CD29 (β1-integrin;f). IMF for CD44 and CD45 revealed the clusters were a heterogeneous population of mesenchymal (CD44;g) and HCs (CD45;h). The clusters resided in close proximity to coronary vessels (i,j) as confirmed by immunostaining on a Tie2Cre;R26R-tdTomato background (k). cv, coronary vessel; ep, epicardium; my, myocardium. Scale bars, 40 μm (a); 20 μm (b–e); 10 μm (f–k). Figure 1: Clusters of cells constrained by ECM exist in the intact adult epicardium. Immunofluorescent staining (IMF) for podoplanin (Pdpn; green) in the intact adult epicardium identifies clusters of cells within basement membrane (white arrowheads; a – c ). Clusters in the epicardium (white arrowheads) are encapsulated by ECM as indicated by IMF for fibronectin (Fn; green; d ). Inset box in d is shown at higher magnification in e , and CD29 (β1-integrin; f ). IMF for CD44 and CD45 revealed the clusters were a heterogeneous population of mesenchymal (CD44; g ) and HCs (CD45; h ). The clusters resided in close proximity to coronary vessels ( i , j ) as confirmed by immunostaining on a Tie2Cre;R26R-tdTomato background ( k ). cv, coronary vessel; ep, epicardium; my, myocardium. Scale bars, 40 μm ( a ); 20 μm ( b – e ); 10 μm ( f – k ). Full size image Epicardial clusters form during early neonatal stages The three-dimensional geometry of the clusters ( Supplementary Movie 1 ) was indicative of tertiary structure within the adult epicardium, over and above the primary cell constituents and secondary two-dimensional organization of the surface epithelium. To determine when this tertiary structure might be established, we focused on early post-natal stages (P) and specifically between days 1 to 7 after birth. This represents a critical window of time on two counts: first, the potential of the epicardium during development is lost at around P4 in terms of an inherent ability of EPDCs to migrate, contribute cardiovascular derivatives and trophic activity [11] , and second, the first week post birth is consistent with loss of regenerative capacity of the heart during P1 to P7. Myocardium was regenerated following ventricular resection injury at P1, but fibrosis and scarring ensued at P7, and although this switch was accounted for by a loss of proliferative potential of resident cardiomyocytes during this time frame, a contribution from a stem/progenitor cell component could not be excluded [12] . At P1, ECM components, such as fibronectin, were expressed widely throughout the heart and there were no apparent distinct clusters of cells within the epicardium ( Fig. 2a ), rather a dispersed incidence of CD44+ and CD45+ cells, which lacked any anatomical constraint ( Fig. 2b,c ). In contrast, by P7 we observed evidence of nascent epicardial ECM, encapsulating small numbers of CD44+ and CD45+ cells ( Fig. 2d–f ). There was no evidence of increased CD44+ or CD45+ cells during this post-natal window, but simply a re-organization into discrete ECM-defined clusters. Thus, the relatively complex epicardial topology appeared to be initiated during the first week after birth, putatively reflecting a more limited stem cell potential, which may in turn contribute to the transient regenerative capacity of the neonatal mouse heart. 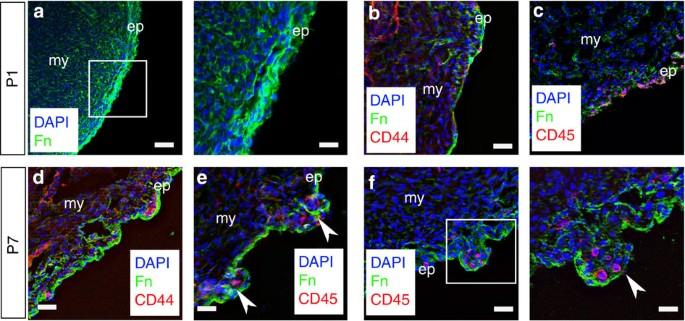Figure 2: Tertiary epicardial structure forms during early post-natal stages. At post-natal day 1 (P1), there is no evidence of cell clusters or higher-order structure in the epicardium; Fn staining is diffused throughout (a), and the CD44+ and CD45+ cells that are present do not occupy discrete locations within the epicardium (b,c). By P7, there is evidence of Fn surrounding the forming clusters containing CD44+ (d) and CD45+ cells (e,f; clusters highlighted by white arrowheads). White inset boxes in the left panels are highlighted at higher magnification in neighbouring right panels. ep, epicardium; my, myocardium. Scale bars,: 50 μm (a, left panel); 20 μm (a, right panel); 30 μm (b–f, left panel); 20 μm (f, right panel). Figure 2: Tertiary epicardial structure forms during early post-natal stages. At post-natal day 1 (P1), there is no evidence of cell clusters or higher-order structure in the epicardium; Fn staining is diffused throughout ( a ), and the CD44+ and CD45+ cells that are present do not occupy discrete locations within the epicardium ( b , c ). By P7, there is evidence of Fn surrounding the forming clusters containing CD44+ ( d ) and CD45+ cells ( e , f ; clusters highlighted by white arrowheads). White inset boxes in the left panels are highlighted at higher magnification in neighbouring right panels. ep, epicardium; my, myocardium. Scale bars,: 50 μm ( a , left panel); 20 μm ( a , right panel); 30 μm ( b – f , left panel); 20 μm ( f , right panel). Full size image A dynamic CD45+ cell and ECM response to ischaemic injury We next determined whether the adult epicardium modulated cell function through structural remodelling under conditions of physiological challenge or pathology [13] . Our focus here was on the novel CD45+ population given the previous description of epicardium-derived CD44-derived mesenchymal stem cell-like cells [9] . MI can cause extensive epicardial fibrosis [14] and, consequently, analyses were carried out on neighbouring intact epicardium, as previously investigated [3] , [4] , [15] . After MI, we observed that resident CD45+ cells began to proliferate at 24 h as detected by pulse chase (injections at 4, 8 and 22 h post MI) with 5-bromo-2'-deoxyuridine (BrdU; Fig. 3a,b ) and co-staining with Ki67 ( Fig. 3c–f ). The numbers of proliferating cells per cluster ranged from 2 to 5 and the mean number of BrdU+ or Ki67+ cells was 3.2±0.6 s.e.m. ( n =15 sections, across 6 hearts at 8 weeks of age). Subsequently, the ECM boundary appeared to break down, within the first 2 days, as best illustrated by a downregulation of fibronectin protein expression leading to loss of epicardial integrity ( Fig. 3g ). ECM breakdown was supported by co-localization of matrix metalloproteinase 2 and 9 expression at corresponding stages post MI ( Supplementary Fig. 2a–d ). This breakdown persisted to day 7 post MI and was accompanied by concomitant expansion of CD45+ cells ( Fig. 3i,k ;) and their release into the subepicardial region and underlying myocardium ( Fig. 3k , right hand panel). Interestingly, regional differences in epicardial response were observed, with disassembly of ECM structures proximal to the site of injury in the left ventricle (LV), whereas those more distal in the right ventricle remained relatively intact, even up to 7 days after injury ( Fig. 3h,j,l ), indicating a spatial gradient in response to injury signalling. After 21 days post MI, the tertiary structure reformed in the LV with restoration of CD44+ cells ( Fig. 3m ) and CD45+ cells ( Fig. 3n ), such that by day 42 there was a return to the pre-injury quiescent state (compare Figs 1a–c and 3o ) and comparable to that observed throughout in the right ventricle ( Fig. 3p ). Collectively, these data suggest that the adult epicardium is a dynamic structure, which responds to injury signals from the infarcted LV to break down the local ECM and release proliferative progenitors into the underlying injured myocardium. 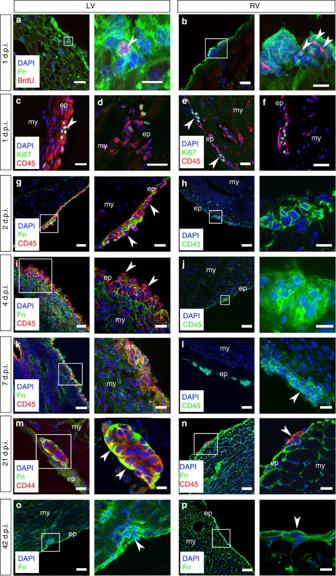Figure 3: Epicardial HC clusters respond dynamically to myocardial injury. Following MI, there is an initial proliferative response as determined by BrdU+ pulse labelling of cluster cells 1 day post injury (1 d.p.i.) in both the left (LV) and right (RV) ventricles (white arrowheads highlight BrdU+ cells;a,b). CD45+ cells located within the epicardial layer were confirmed as undergoing cell cycle activity via Ki67 co-staining in both the LV (c,d) and RV (e,f; white arrowheads highlight CD45+/Ki67+ cells). As early as day 2 post MI (2 d.p.i.) in the LV, the clusters begin to break down (g). Disassembly of ECM-encapsulated cell clusters persists through day 4 (4 d.p.i.;i) and progresses to day 7 (7 d.p.i.;k) to release CD45+ cells (g,i,k) This is not the case in the RV where the clusters remain intact over the same time course of injury constraining the resident cell types (h,j,l); white arrowhead inlhighlights intact cluster 7 d.p.i. By day 21 post MI (21 d.p.i.), the clusters have reformed (white arrowheads in higher magnification view highlight Fn at the apical surface) in the LV (m) to resemble the persistent intact clusters of the RV (n) and pre-injury state (Fig. 1); the reinstated ‘niche’ is evident 42 days post MI (42 d.p.i.;o) and is comparable to that in the RV as highlighted by white arrowheads (p). White inset boxes in the left panels are highlighted at higher magnification in neighbouring right panels. ep, epicardium; my, myocardium. Scale bars, 50 μm (a–p, left panels); 20 μm (g,i,j,l,n); 10 μm (a,b,h,k,m–p, right panels). Figure 3: Epicardial HC clusters respond dynamically to myocardial injury. Following MI, there is an initial proliferative response as determined by BrdU+ pulse labelling of cluster cells 1 day post injury (1 d.p.i.) in both the left (LV) and right (RV) ventricles (white arrowheads highlight BrdU+ cells; a , b ). CD45+ cells located within the epicardial layer were confirmed as undergoing cell cycle activity via Ki67 co-staining in both the LV ( c , d ) and RV ( e , f ; white arrowheads highlight CD45+/Ki67+ cells). As early as day 2 post MI (2 d.p.i.) in the LV, the clusters begin to break down ( g ). Disassembly of ECM-encapsulated cell clusters persists through day 4 (4 d.p.i. ; i ) and progresses to day 7 (7 d.p.i. ; k ) to release CD45+ cells ( g , i , k ) This is not the case in the RV where the clusters remain intact over the same time course of injury constraining the resident cell types ( h , j , l ); white arrowhead in l highlights intact cluster 7 d.p.i. By day 21 post MI (21 d.p.i. ), the clusters have reformed (white arrowheads in higher magnification view highlight Fn at the apical surface) in the LV ( m ) to resemble the persistent intact clusters of the RV ( n ) and pre-injury state ( Fig. 1 ); the reinstated ‘niche’ is evident 42 days post MI (42 d.p.i. ; o ) and is comparable to that in the RV as highlighted by white arrowheads ( p ). White inset boxes in the left panels are highlighted at higher magnification in neighbouring right panels. ep, epicardium; my, myocardium. Scale bars, 50 μm ( a – p , left panels); 20 μm ( g , i , j , l , n ); 10 μm ( a , b , h , k , m – p , right panels). Full size image Canonical Wt1+ epicardial cells are distinct from HC clusters We next investigated the relative spatial localization of reactivated Wt1+ cells, previously identified as an important subpopulation of epicardial progenitors following MI [3] , [4] , within the higher-order structure of the adult epicardium. Injury-activated Wt1+ cells were distinct from the resident CD45+ HC population ( Fig. 4a,b ) and, although they were not localized within the clusters they resided immediately proximal ( Fig. 4c,d ). The response of the Wt1+ population varied considerably depending on the extent of infarction and injury, as previously reported [3] , [4] . Following injury (day 4 post MI), the breakdown of the ECM clusters and expansion of the sub-epicardial region contained some Wt1+ cells, as reported by Wt1CreERT2;R26R-tdTomato lineage tracing from developmental stages alongside immunostaining for Wt1 ( Fig. 4e,f ). Efficient recombination of the R26R-tdTomato, by tamoxifen-induced Wt1CreERT2, was observed with specific tdTomato+ reporter labelling of the epicardium throughout development and into adulthood ( Supplementary Fig. 3a–l ), as well as efficient tracing of Wt1+ cell derivatives, such as smooth muscle cells, within the adult heart ( Supplementary Fig. 4a–d ). Wt1-tdTomato+ cells were also evident throughout the myocardium ( Fig. 4e ), reflecting the increased contribution of Wt1 derivatives over time ( Supplementary Fig. 3h–l ). The Wt1-negative cells in the sub-epicardial region were predominantly CD45+ ( Fig. 4g,h ), suggesting an influx of HCs consistent with an early pro-inflammatory response [16] . The extent of CD45+ cellular contribution to the expanded epicardium at day 4 post MI was comparable to that observed within the bone marrow ( Supplementary Fig. 5 ). 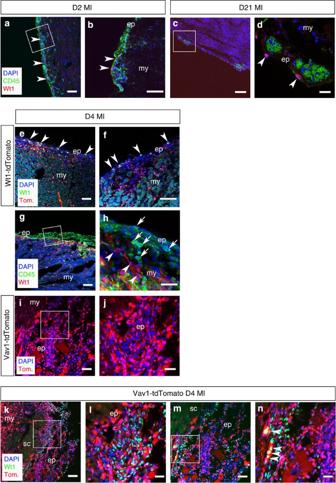Figure 4: Injury-activated Wt1+ epicardial cells are mutually exclusive from CD45/Vav1+ HCs in the expanded epicardium. At 2 days post MI (D2 MI), cells re-expressing Wt1 (highlighted by white arrowheads) are distinct from the CD45+ population residing in the expanding epicardium (a,b; white inset box ina, shown at higher magnification inb). At day 21 post MI (D21 MI), Wt1 cells reside proximal to the niche-like clusters (c,d; white inset box inc, shown at higher magnification ind). Wt1CreERT2;R26R-tdTomato labelling and Wt1-antibody staining revealed Wt1+/tdTomato+ cells residing in the expanded epicardium and tdTomato-labelled derivatives within the underlying myocardium (e,f; arrowheads indicate double-positive Wt1+/tdTomato+ cells) relative to an abundance of infiltrating CD45+ cells (g,h; white inset box ingshown in higher magnification inh; arrows inhindicate CD45+ cells and arrowheads indicate Wt1+ cells) and HCs labelled in a Vav1-Cre; R26R-tdTomato reporter line (i,j; white inset box ini, shown at higher magnification inj). At day 4 post MI (D4 MI), Wt1 and tdTomato are expressed in distinct cell populations with a few notable exceptions highlighted by white arrowheads (k–n; white inset boxes inkandmare highlighted at higher magnification inlandn,respectively). ep, epicardium; my, myocardium; sc, scar. Scale bars, 50 μm, (a,c,e,g,i); 100 μm (k,m); 20 μm (b,d); 30 μm (f,h,j,l,n). Figure 4: Injury-activated Wt1+ epicardial cells are mutually exclusive from CD45/Vav1+ HCs in the expanded epicardium. At 2 days post MI (D2 MI), cells re-expressing Wt1 (highlighted by white arrowheads) are distinct from the CD45+ population residing in the expanding epicardium ( a , b ; white inset box in a , shown at higher magnification in b ). At day 21 post MI (D21 MI), Wt1 cells reside proximal to the niche-like clusters ( c , d ; white inset box in c , shown at higher magnification in d ). Wt1CreERT2;R26R-tdTomato labelling and Wt1-antibody staining revealed Wt1+/tdTomato+ cells residing in the expanded epicardium and tdTomato-labelled derivatives within the underlying myocardium ( e , f ; arrowheads indicate double-positive Wt1+/tdTomato+ cells) relative to an abundance of infiltrating CD45+ cells ( g , h ; white inset box in g shown in higher magnification in h ; arrows in h indicate CD45+ cells and arrowheads indicate Wt1+ cells) and HCs labelled in a Vav1-Cre; R26R-tdTomato reporter line ( i , j ; white inset box in i , shown at higher magnification in j ). At day 4 post MI (D4 MI), Wt1 and tdTomato are expressed in distinct cell populations with a few notable exceptions highlighted by white arrowheads ( k – n ; white inset boxes in k and m are highlighted at higher magnification in l and n, respectively). ep, epicardium; my, myocardium; sc, scar. Scale bars, 50 μm, ( a , c , e , g , i ); 100 μm ( k , m ); 20 μm ( b , d ); 30 μm ( f , h , j , l , n ). Full size image CD45+ epicardial cells arise from the haemagenic endothelium To confirm a haematopoietic origin for the CD45+ population, we traced cells residing in the sub-epicardium using Vav1-Cre; R26R-tdTomato mice. Vav1-Cre labels developmental haematopoietic progenitors arising from the yolk sac blood islands ( Supplementary Fig. 6a,b ) and the aorta-gonad-mesonephros region (sites of primitive and definitive haematopoiesis, respectively; Supplementary Fig. 6c ), the fetal liver (a second site of definitive haematopoiesis; Supplementary Fig. 6d,e ), as well as adult pan-circulatory HCs [17] , [18] , [19] . Significant numbers of Vav1-tdTomato+ cells were observed in the expanded sub-epicardium ( Fig. 4i,j ) by day 4 post MI and these were largely negative for Wt1 protein expression aside from isolated examples of tdTomato+/Wt1+ cells ( Fig. 3k–n ). The relative proportion of single tdTomato+ (Vav1+) versus single Wt1+ cells was 77.6±16.3% versus 22.4±4.8% (mean %±s.e.m. ; P ≤0.001; n =6 hearts; Student’s t -test). Importantly, we excluded the endothelial markers, CD31 and Endomucin, from the CD45+ sub-population located within the epicardial and sub-epicardial regions at day 4 post MI, in support of an HC phenotype ( Supplementary Fig. 7a–c ). Given the prevalence of CD45+ and Vav1+ cells in both the intact epicardium and in response to injury, we traced Vav1-tdTomato+ cells through developmental stages to determine whether there may be an embryonic haematopoietic contribution to the forming epicardium ( Fig. 5 ). We observed tdTomato+ cells residing in the epicardium and underlying myocardium from E12.5, with a prominent contribution at both E14.5 ( Fig. 5a,b ) and E16.5 ( Fig. 5c,d ). The presence of HCs within the embryonic epicardium was confirmed by immunostaining for CD45 at E14.5 in Vav1-Cre;R26R-tdTomato mice ( Fig. 5e–h ), which revealed CD45+/m-tomato+ cells integrated within the outer epicardial layer ( Fig. 5f–h ) that were negative for the endothelial cell marker CD31 ( Supplementary Fig. 7d ). Not all Vav1+ cells were CD45+, consistent with the broader Vav1+ lineage [17] , but all CD45+ cells localized within the epicardium were Vav1+, as evident in the lineage-traced hearts at E14.5 ( Fig. 5f–h ). At higher magnification ( Fig. 5g ), the CD45+/tdTomato+ cells were located on the apical surface of the heart, contiguous with the outer epicardium, suggesting they contributed intrinsically to the polarized epithelium. In contrast, immunostaining for CD45 in Wt1CreERT2;R26R-tdTomato mice ( Fig. 5i–l ), revealed that the HCs were distinct from Wt1-tdTomato+ epicardial cells ( Fig. 5l ). The incidence of CD45+ cells residing in the epicardium significantly increased from 7.9±0.01% at E12.5 to a maximum of 17.0± 1.2% at E14.5 ( P ≤0.001; n =6 hearts; Student’s t -test; Fig. 5m ). To exclude the possibility that the CD45+ cells might have arisen from the PEO ( Fig. 5n ), we stained Vav1-tdTomato mice with α-CD45 and observed that both tdTomato and CD45 were not expressed within the Wt1+ PEO ( Fig. 5o,p ). In addition, lineage tracing with Gata5Cre;R26R-tdTomato and Wt1CreERT2;R26R-tdTomato mice revealed that neither Gata5+ nor Wt1+ epicardial lineages gave rise to CD45 cells ( Supplementary Fig. 8 ). In contrast, a proportion of Gata5-tdTomato+ cells (<10%) were also CD44+, consistent with a mesenchymal-like cell origin from the PEO [9] . These data suggest that HCs contribute to the forming epicardium during development and arise from a Vav1+ haemogenic (haemangiogenic) source, which is distinct from the PEO. 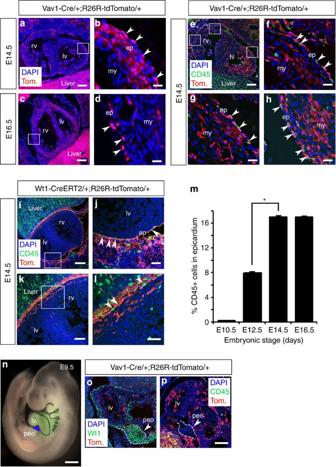Figure 5: Vav1+/CD45+ HCs contribute to the developing epicardium and do not originate from the PEO. In Vav1-Cre;R26R-tdTomato embryonic hearts, tdTomato+ (Vav1+) haematopoietic stem cells (HSCs) contribute to the developing epicardium from E12.5 to E16.5. At E14.5 (a,b) and E16.5 (c,d), tdTomato+ (Tom) cells reside in the epicardium and underlying myocardium (white inset boxes inaandcare highlighted at higher magnification inbandd, respectively; white arrowheads inbanddhighlight tdTomato+ cells specifically in the epicardium). At E14.5, further immunostaining for combined α-CD45+ and tdTomato (e) revealed that all CD45+ cells residing within the developing epicardium were Vav1-tdTomato+ (f–h; white arrowheads highlight double-positive cells), whereas Vav1-tdTomato+ cells negative for CD45+ were localized within the underlying myocardium (f–h). The CD45+ HCs were distinct from the Wt1+ contribution as indicated by CD45+ immunostaining in conjunction with lineage tracing in WtCreERT2;R26R-tdTomato developing hearts at E14.5 (i–l; white inset boxes iniandkare highlighted at higher magnification injandl, respectively; white arrowheads injandlhighlight CD45+ cells specifically in the epicardium). The number of CD45+ cells that contributes to the epicardium increases from E10.5, coincident with formation of the epicardium, through to E16.5 with a significant increase between E12.5 and 14.5 (mean % CD45+ cells ± s.e.m.;P≤0.001;n=6 hearts;m). In Vav1-tdTomato-labelled embryos, tdTomato+ cells do not contribute to the proepicardial organ (peo; indicated in blue inn; rest of heart indicated in green via Nkx2.5Cre;R26R-EYFP) at E9.5 (o; peo is demarcated by Wt1 immunostaining) and CD45+ cells do not localize to the peo (p), suggesting tdTomato/CD45+ HCs that contribute to the forming epicardium arise from an alternate source, previously described as the haemagenic endothelium and/or fetal liver (Supplementary Fig. 6). ep, epicardium; lv, left ventricle; my, myocardium; peo, proepicardial organ; rv, right ventricle. Scale bars, 200 μm (a,i); 20 μm (b,d,f–h); 400 μm (c,e); 50 μm (j,l); 100 μm (i,o,p); 600 μm (n). All statistics are calculated by Studentst-test; *P≤0.001. Figure 5: Vav1+/CD45+ HCs contribute to the developing epicardium and do not originate from the PEO. In Vav1-Cre;R26R-tdTomato embryonic hearts, tdTomato+ (Vav1+) haematopoietic stem cells (HSCs) contribute to the developing epicardium from E12.5 to E16.5. At E14.5 ( a , b ) and E16.5 ( c , d ), tdTomato+ (Tom) cells reside in the epicardium and underlying myocardium (white inset boxes in a and c are highlighted at higher magnification in b and d , respectively; white arrowheads in b and d highlight tdTomato+ cells specifically in the epicardium). At E14.5, further immunostaining for combined α-CD45+ and tdTomato ( e ) revealed that all CD45+ cells residing within the developing epicardium were Vav1-tdTomato+ ( f – h ; white arrowheads highlight double-positive cells), whereas Vav1-tdTomato+ cells negative for CD45+ were localized within the underlying myocardium ( f – h ). The CD45+ HCs were distinct from the Wt1+ contribution as indicated by CD45+ immunostaining in conjunction with lineage tracing in WtCreERT2;R26R-tdTomato developing hearts at E14.5 ( i – l ; white inset boxes in i and k are highlighted at higher magnification in j and l , respectively; white arrowheads in j and l highlight CD45+ cells specifically in the epicardium). The number of CD45+ cells that contributes to the epicardium increases from E10.5, coincident with formation of the epicardium, through to E16.5 with a significant increase between E12.5 and 14.5 (mean % CD45+ cells ± s.e.m. ; P ≤0.001; n =6 hearts; m ). In Vav1-tdTomato-labelled embryos, tdTomato+ cells do not contribute to the proepicardial organ (peo; indicated in blue in n ; rest of heart indicated in green via Nkx2.5Cre;R26R-EYFP) at E9.5 ( o ; peo is demarcated by Wt1 immunostaining) and CD45+ cells do not localize to the peo ( p ), suggesting tdTomato/CD45+ HCs that contribute to the forming epicardium arise from an alternate source, previously described as the haemagenic endothelium and/or fetal liver ( Supplementary Fig. 6 ). ep, epicardium; lv, left ventricle; my, myocardium; peo, proepicardial organ; rv, right ventricle. Scale bars, 200 μm ( a , i ); 20 μm ( b , d , f – h ); 400 μm ( c , e ); 50 μm ( j , l ); 100 μm ( i , o , p ); 600 μm ( n ). All statistics are calculated by Students t -test; * P ≤0.001. Full size image Bone marrow-derived HCs integrate into the adult epicardium To explore a potential haematopoietic contribution to the epicardium of the intact heart during adult homeostasis, we carried out cell transplantation of either labelled bone marrow (BM) from β-actin-Cre;R26R-EYFP or HCs from Vav1-Cre;R26R-tdTomato donors into lethally or sub-lethally irradiated unlabelled hosts ( Supplementary Fig. 9a,b ). Ionizing radiation targets mitotically active cells, which in the intact adult epicardium are likely to be represented by the previously described CD44+ cCFU-Fs [9] . Haematopoietic reconstitution occurs in mouse in waves, with transient reconstituting cells detectable after 2–4 weeks, but which disappear after 8–10 weeks, and longer-term reconstituting cells that contribute at least 6 months after transplantation [20] . Thus, a 6-month follow-up herein was employed to negate the possibility of HC influx due to irradiation-induced inflammation and, consequently, to investigate potential long-term (homeostatic) BM contribution and epicardial cell turnover. Following irradiation, we were unable to detect either CD44+ cells, consistent with ablation of the cCFU-Fs as previously described [9] or host CD45+ cells, even after 6 months. YFP+ BM cells were observed in the epicardium and sub-epicardial region after 2 months, residing both within the single epicardial cell layer overlying the myocardium and epicardial cell clusters ( Fig. 6a–d ). YFP+ cells were also observed to traffic into adult epicardial clusters at 2 months ( Supplementary 10a,b ). At 6 months, a YFP+ contribution was still evident in the epicardium with some contribution to the adjacent myocardium ( Fig. 6e–h ). Quantitation revealed the overall numbers of YFP+ BM cells significantly increased in the epicardium over the 4-month duration of the analyses ( P ≤0.001; n =6 hearts; Student’s t -test; Fig. 6i ). Although early on, following host γ-irradiation, donor BM-derived cells may infiltrate due to radiation-induced injury and inflammation, the significant YFP+ BM presence at 6 months represents an injury-independent contribution. Podoplanin immunostaining confirmed the localization of YFP+ BM derivatives to the epicardium at both 2 and 6 months ( Fig. 6j,n ); although there was significant variation in the abundance of transplanted cells depending on location within the chambers (compare Fig. 6k,m with Fig. 6n,q ), after 2 and 6 months. The YFP+ cells were all CD45+ indicative of the HC compartment of the BM inoculum ( Fig. 6k,o ). The majority of those residing within the epicardium itself (>90%) were negative for the monocyte marker Ly-6C ( Fig. 6l,p ); however, a more detailed characterization of their immuno-phenotype revealed a minor subpopulation (<10%) of transplanted tomato+/CD45+ cells, which were positive for the macrophage marker F4/80 ( Supplementary Fig. 11a,b ); in contrast, none of the transplanted cells co-stained for the neutrophil marker myeloperoxidase ( Supplementary Fig. 11c ). Evidence of subsequent YFP+ BM cell differentiation within the myocardium was observed by virtue of cells co-staining for the pericyte marker NG2+ ( Fig. 6m,q ; Supplementary Fig. 12a ). Further analyses on the lineage potential of the transplanted BM cells at 2 months revealed co-staining of YFP+ cells with an additional pericyte marker CD146 (ref. 21 ( Supplementary Fig. 12b ) and the exclusion of the fibroblast marker PDGFRβ Supplementary Fig. 12c,d ). 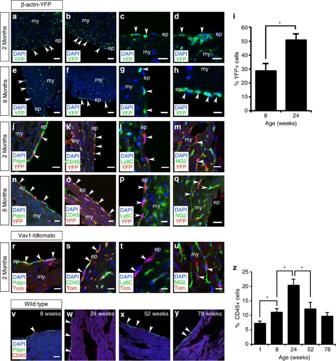Figure 6: Bone marrow transplantation reveals a haematopoietic contribution to the adult epicardium that alters with age. Two months after whole bone marrow (BM) transplantation of β-actin-Cre;R26R-EYFP labelled BM into lethally irradiated unlabelled hosts (Supplementary Fig. 9a), YFP+ cells are localized to the adult epicardium (a,b; as highlighted by white arrowheads) and the YFP+ BM cells contribute to epicardial clusters (c,d). The YFP+ cells persist at 6 months post transplantation and are localized to the epicardium (e–h; as highlighted by white arrowheads) and there was a significant increase in epicardial YFP+ cells over the intervening 4 months (mean %YFP+ cells ± s.e.m.;P≤0.001;n=6 hearts;i). At 2 and 6 months, podoplanin immunostaining confirmed the epicardial localization of YFP+ BM cells (j,n) and these were CD45+ (k,o; white arrowheads; white asterisk highlights a YFP+/CD45− cell), suggesting they represented the haematopoietic compartment of the whole BM inoculum, but were negative for Ly6C, thus excluding the mature myeloid lineage (l,p; white arrowheads indicate YFP+ cells in red which do not co-express Ly6C in green). A sub-population of YFP+ BM cells within the underlying myocardium expressed NG2, suggesting they had differentiated into pericytes (m,q; highlighted by white arrowheads). Two months after transplantation of flow-sorted Vav1+ cells, from Vav1-Cre;R26R-tdTomato-labelled bone marrow into lethally irradiated unlabelled hosts (Supplementary Fig. 9b), tdTomato+ cells are localized to the podoplanin+ adult epicardium (r; as highlighted by white arrowheads). The tdTomato+ BM cells were CD45+ (s; white arrowheads), confirming them as representative of the haematopoietic compartment of the whole BM inoculum. The tdTomato+ donor cells were negative for Ly6C, thus excluding the mature myeloid lineage (t; white arrowheads indicate tdTomato+ cells in red, which do not co-express Ly6C in green). A sub-population of tdTomato+ BM cells within the underlying myocardium expressed NG2, suggesting they had differentiated into pericytes (u; highlighted by white arrowheads). The number of CD45+ cells increased in the adult epicardium with age up to 24 weeks (v,w) but decreased thereafter as measured at 52 and 78 weeks (x,y). The increases between 1 and 8, and 8 and 24 weeks were significant, as was the decrease between 24 and 52 weeks (mean % CD45+ cells±s.e.m. ofn=3 hearts, 6 sections analysed per heart;P≤0.001;z), suggesting an increased haematopoietic epicardial reserve with adulthood to maturity but depletion or impaired replenishment with advanced age (12 and 18 months). ep, epicardium; my, myocardium. Scale bars, 50 μm (a,b,e,f,v–y); 20 μm (c,d,j,k–o,q–s,u); 10 μm; (g,h); 10 μm (i,p,t). All statistics are calculated by Student’st-test; *P≤0.001. Figure 6: Bone marrow transplantation reveals a haematopoietic contribution to the adult epicardium that alters with age. Two months after whole bone marrow (BM) transplantation of β-actin-Cre;R26R-EYFP labelled BM into lethally irradiated unlabelled hosts ( Supplementary Fig. 9a ), YFP+ cells are localized to the adult epicardium ( a , b ; as highlighted by white arrowheads) and the YFP+ BM cells contribute to epicardial clusters ( c , d ). The YFP+ cells persist at 6 months post transplantation and are localized to the epicardium ( e – h ; as highlighted by white arrowheads) and there was a significant increase in epicardial YFP+ cells over the intervening 4 months (mean %YFP+ cells ± s.e.m. ; P ≤0.001; n =6 hearts; i ). At 2 and 6 months, podoplanin immunostaining confirmed the epicardial localization of YFP+ BM cells ( j , n ) and these were CD45+ ( k , o ; white arrowheads; white asterisk highlights a YFP+/CD45− cell), suggesting they represented the haematopoietic compartment of the whole BM inoculum, but were negative for Ly6C, thus excluding the mature myeloid lineage ( l , p ; white arrowheads indicate YFP+ cells in red which do not co-express Ly6C in green). A sub-population of YFP+ BM cells within the underlying myocardium expressed NG2, suggesting they had differentiated into pericytes ( m , q ; highlighted by white arrowheads). Two months after transplantation of flow-sorted Vav1+ cells, from Vav1-Cre;R26R-tdTomato-labelled bone marrow into lethally irradiated unlabelled hosts ( Supplementary Fig. 9b ), tdTomato+ cells are localized to the podoplanin+ adult epicardium ( r ; as highlighted by white arrowheads). The tdTomato+ BM cells were CD45+ ( s ; white arrowheads), confirming them as representative of the haematopoietic compartment of the whole BM inoculum. The tdTomato+ donor cells were negative for Ly6C, thus excluding the mature myeloid lineage ( t ; white arrowheads indicate tdTomato+ cells in red, which do not co-express Ly6C in green). A sub-population of tdTomato+ BM cells within the underlying myocardium expressed NG2, suggesting they had differentiated into pericytes ( u ; highlighted by white arrowheads). The number of CD45+ cells increased in the adult epicardium with age up to 24 weeks ( v , w ) but decreased thereafter as measured at 52 and 78 weeks ( x , y ). The increases between 1 and 8, and 8 and 24 weeks were significant, as was the decrease between 24 and 52 weeks (mean % CD45+ cells±s.e.m. of n =3 hearts, 6 sections analysed per heart; P ≤0.001; z ), suggesting an increased haematopoietic epicardial reserve with adulthood to maturity but depletion or impaired replenishment with advanced age (12 and 18 months). ep, epicardium; my, myocardium. Scale bars, 50 μm ( a , b , e , f , v – y ); 20 μm ( c , d , j , k – o , q –s, u ); 10 μm; ( g , h ); 10 μm ( i , p , t ). All statistics are calculated by Student’s t -test; * P ≤0.001. Full size image Transplanted Vav1+ CD45+ cells become depleted with age The BM findings were supported by transplantation with lineage-negative HCs as labelled by Vav1-Cre;R26R-tdTomato. Tomato+ cells were observed in the epicardium at 2 months as demarcated by podoplanin ( Fig. 6r ) and were localized into clusters ( Supplementary Fig. 10b ). These cells were CD45+, and consistent with the whole BM YFP+ transplantation data the majority were Ly-6C− ( Fig. 6s,t ), of which a proportion had differentiated into NG2+ pericytes located in the underlying myocardium ( Fig. 6u ), consistent with the previous observations for whole BM. Tomato+ cells post-BM transplantation either residing within the epicardial or underlying myocardium were also negative for the endothelial cell markers CD31 and Endomucin ( Supplementary Fig. 7e–h ). We subsequently investigated the status of the CD45+ compartment in older animals, given that aging is proposed to act as a negative modifier of cellular efficacy (reviewed in ref. 22 ). A time course from post-natal day 7 (P7) through to 18 months suggested the epicardium is turned over via HC contribution, with increasing recruitment of CD45+ cells between P7 and 6 months ( Fig. 6v–y ). In older mice, the number of CD45+ cells was significantly reduced from 20.3±2.1% at 6 months down to 12.2±2.2% at 12 months and 9.67±1.3% at 18 months (mean±s.e.m. of n =3 hearts, 6 sections analysed per heart; P ≤0.001; Student’s t -test; Fig. 6z ), suggesting that either HC contribution to the epicardium is compromised with age or the resident CD45+ population is depleted over time. The characterization of the adult epicardium as a complex anatomical structure is in stark contrast to the widely held view of the epicardium as a simple mesothelium and single cell layer epithelium. The adult epicardial topology contained features associated with a canonical stem cell niche, as have been characterized in the BM, skin (hair follicle bulge), intestine (villi and crypts) and subventricular zone of the brain [23] , [24] , [25] , [26] . Most notably, the existence of clusters of cells, within the epicardium, encased by basement membrane and with associated vascular support meets several anatomical niche criteria (reviewed in ref. 27 ). In the adult heart, cell turnover and renewal based on stem cell deployment has been demonstrated [9] , [28] ; yet, occupancy of a cardiogenic stem cell niche [29] remains to be determined [30] , [31] . Whether the epicardium can be regarded as a classical niche requires functional disruption of the ‘microenvironment’ described, so as to directly affect the resident stem/progenitor cell population in terms of homing, multipotency or differentiation of progeny during homeostasis or injury. These represent ongoing, but technically challenging, experiments that lie outside the scope of the current study. The ‘niche-like’ structure is formed during a critical post-natal window when the inherent regenerative capacity of the heart is lost within the first week after birth [12] , [32] . This may reflect the limited reparative capacity of the maturing heart, at least in part, via the constraint of epicardial cells within the ECM ( Supplementary Movie 1 ). Following myocardial injury, an initial breakdown of epicardial basement membrane was accompanied by release of constituent cells and subsequent reformation via assembly of ECM. The ECM plays a key role in a niche setting, as it is thought to ‘protect’ the progenitor compartment from depletion while simultaneously protecting the host tissue from overproliferation. Although the resident cells remain in a state of quiescent under normal conditions, the ECM is also important for transmitting signals to induce self-renewal and/or differentiation during physiological stress or in response to injury (reviewed in ref. 33 ). The resident cellular compartments in the epicardium consist of both CD44+ mesenchymal-like stem cells (cCFU-Fs), previously demonstrated to be of epicardial origin [9] , and a novel BM-derived CD45+ haematopoietic population, which appeared to participate in homeostatic EPDC turnover with age. Both cell types are incorporated into the clusters irrespective of origin during the first week of life and the CD45+ population is subsequently replenished from BM. Although tissue monocytes of BM origin are known to migrate into almost every solid organ of the body, including the adult heart (reviewed in ref. 34 ), an HC contribution to the epicardium represents a novel finding. The contribution to adult epicardium by HCs was injury independent, with long-term reconstitution of donor HCs following BM transplantation well beyond any potential inflammatory response arising from host irradiation. Although we were unable to definitively discriminate the response of a resident CD45+/Vav1+ population from BM infiltration during injury, the remodelling of the ECM surrounding the cell clusters and resident CD45+ cell proliferation was distinct from an influx of BM HCs post MI. Moreover, the long-term reconstitution of BM/Vav1+ transplanted cells suggested the BM can act as a source of replenishment of epicardial HCs, which in turn are then able to respond to injury independently of an acute BM response. Previously, whole BM transplantation revealed that engraftment of BM-derived cells occurred as part of normal cardiac valve function, setting a precedent for a BM contribution to cardiovascular homeostasis per se [35] . Our study supports a role for BM in adult heart homeostasis and the HC turnover, contrasts with the current steady-state view of a single source of epicardium maintained throughout adulthood; this in turn reinforces the concept that the adult mammalian heart should no longer be considered a post-mitotic organ [36] , [37] , [38] . CD45+ HCs were labelled by a Vav1-Cre-induced reporter, which, when subsequently traced through developmental stages, revealed a novel contribution to the embryonic epicardium from the haemagenic endothelium or fetal liver [18] , [19] . A distinct sub-population of HCs was recently characterized within the developing heart as arising from the endocardial lineage, and contributing an additional reservoir for definitive haematopoiesis [39] . In contrast, we report here the integration of CD45+ HCs into the developing epicardium, arising from classical sites of both primitive (yolk sac blood islands) and definitive (aorta-gonad-mesonephros, fetal liver) haematopoiesis within the embryo. Notably, the CD45+/Vav1+ population was entirely distinct from Wt1-expressing cells of the PEO. Cellular heterogeneity within the epicardium has been reported in previous studies, which focused on the lineage composition of the PEO, as the canonical source of epicardium progenitors [9] , [40] , [41] . Although a number of sub-compartments within the PEO itself have been well characterized, notably those labelled as Wt1+ and Tbx18+, as well as partially overlapping Sema3D+ and Scleraxis+ sub-populations [40] , a novel source of epicardial cells of alternate embryological origin has not hitherto been reported. Our findings challenge current dogma that the epicardium arises exclusively from the transient, mesoderm-derived PEO, located at the inflow region of the developing heart [5] . Understanding the developmental biology of the epicardium is instrumental for developing novel cell therapies for heart regeneration. We and others have previously demonstrated that the adult epicardium, can be reactivated, via induction of an embryonic gene programme, to act as a potential resident cell source, which can be tapped to reconstitute damaged heart tissue [2] , [3] , [4] , [7] , [42] . This potential of the adult epicardium was realized entirely in the context of a homogeneous Wt1+ epicardial cell response. The integral contribution of CD45+ HCs to both embryonic and adult epicardium, and the turnover of a BM-derived HC source during adult homeostasis, should yield important insight into the potential for both self-renewal and resident cell-based repair within the heart. It will be of interest to determine whether the HC contribution to the epicardium and complex tertiary structure of constraining ECM identified here in mouse translates to humans, and whether it might be targeted for activation and contribution to tissue regeneration following ischaemic heart disease. Generation of epicardial trace mice Wt1 CreERT2/+ , Gata5 Cre/+ and Vav1 Cre/+ ; R26R tdTomsto/+ mice were generated crossing Rosa26R-tdTomato [43] reporter mice with Wt1 CreERT2/+ (ref. 44 ), Gata5 Cre/+ (ref. 45 ) and Vav1 Cre/+ (ref. 46 ) mice, and genotyping as previously described. Wt1 expression in the developing epicardium was achieved through double intraperitoneal tamoxifen injections. Toxic effects of tamoxifen were countered by co-injection of progesterone. Pregnant dams received two 2-mg tamoxifen injections and simultaneous 1 mg progesterone injections at E9 and E11. Embryos were collected at specific time points and prepared for immunofluorescence. Images were obtained using a using Zeiss LSM 710 confocal microscope equipped with argon and helium neon lasers using × 20, × 40 and × 63/1.4 (oil immersion) objectives. All animal experiments were carried out according to the UK Home Office project licences PPL30/2987 Compliant with the UK Animals (Scientific Procedures) Act 1986 and approved by the University College London Biological Services Ethical Review Process. Animal husbandry at UCL Biological Services was in accordance with the UK Home Office Certificate of Designation. Immunodetection Immunofluorescence was performed on cryosections of embryonic, uninjured and post-MI hearts using standard protocols with the following antibodies: green fluorescent protein (GFP; Clontech and Abcam, which detect EYFP), Fibronectin, CD44, CD45, BrdU, Hyaluronic acid, Ly-6C and Wt1 (all from Abcam), podoplanin (Novus Europe), Collagen IV (AbD Serotec), NG2 (Chemicon) and CD29 (Millipore). To rule out the possibility of autofluorescence accounting for the detection of either GFP or yellow fluorescent protein (YFP) protein expression, sections through the LV were stained with a polyclonal anti-GFP antibody (which detects both fluorescent proteins). The specificity of the anti-GFP antibody was ascertained by immunofluorescence on non-primed, intact hearts, which detected neither labelled cells in the epicardial region, nor their derivatives (no signal). To detect BrdU-positive nuclei, sections were treated with 2 N HCl for 30 min at room temperature (22 °C) to denature the DNA, and neutralized in 0.1 M sodium borate pH 8.5 for 12 min before incubation with the anti-BrdU antibody. Owing to the destruction of cellular antigens resulting from acid treatment, these steps were performed after the incubation with antibodies to GFP and SαA. Images were acquired using a Zeiss LSM 710 confocal microscope equipped with argon and helium neon lasers using × 20, × 40 and × 63/1.4 (oil immersion) objectives. mTomato fluorescent protein used to test the Cre-lox recombination of Gata5 , Wt1 and Vav1 Cre driver strains was visualized directly without secondary staining protocols at its emission wavelength of 581 nm. MI surgery Mice were housed and maintained in a controlled environment. All surgical and pharmacological procedures were performed in accordance with the Animals (Scientific Procedures) Act 1986, (Home Office, UK). MI was induced in isoflurane-anaesthetized mice by permanent ligation of the left anterior descending artery. On recovery, animals received intraperitoneal injection of BrdU (80 mg kg −1 ; Invitrogen) if required. Further injections were administered at 2, 4 and 8 h post surgery. Hearts were harvested at 2, 4, 7, 21 and 42 days after ligation and bisected transversely midway through the scar and fixed in 4% paraformaldehyde for cryosectioning and immunostaining analyses. BM collection All mice were culled before tissue dissection in accordance with the Home Office regulation. Hind limbs were dissected to isolate the femur and knee joint. Femurs were flushed using a 23-G needle and 1-ml syringe (both from Becton Dickinson) with PBS, and cells were collected and kept on ice. Cells were then filtered using a 70-μm cell strainer (Becton Dickinson) and centrifuged at 200 g for 5 min. Five millilitres of Red Cell Lysis Buffer was used to resuspend the pellet and incubated for 3 min before centrifuging at 200 g for 5 min to pellet the cells. Cells were then used for RNA extraction or transplantation. BM irradiation and transplantation Mice are housed and maintained in a controlled environment. All procedures are performed in accordance with the Animals (Scientific Procedures) Act 1986, (Home Office, UK). Mice were sub-lethally (6 Gy) irradiated or lethally irradiated, using split dose (4+5 Gy) radiation, 24 h before cell transfer. Donor mice were culled before tissue dissection in accordance with the Home Office regulation. Hind limbs were dissected to isolate the femur and tibia bones. Single-cell suspensions were isolated in Hepes-buffered HBSS and either transplanted directly into recipient mice or lineage-negative cells were first purified using the mouse Lineage Cell Depletion kit (Miltenyi Biotec). In total, 1 × 10 7 or 2.5 × 10 5 lineage-negative cells were injected via the lateral tail vein. How to cite this article: Balmer, G. M. et al. Dynamic haematopoietic cell contribution to the developing and adult epicardium. Nat. Commun. 5:4054 doi: 10.1038/ncomms5054 (2014).